The central role of EED in the orchestration of polycomb group complexes Polycomb repressive complexes 1 and 2 (PRC1 and 2) play a critical role in the epigenetic regulation of transcription during cellular differentiation, stem cell pluripotency and neoplastic progression. Here we show that the polycomb group protein EED, a core component of PRC2, physically interacts with and functions as part of PRC1. Components of PRC1 and PRC2 compete for EED binding. EED functions to recruit PRC1 to H3K27me3 loci and enhances PRC1-mediated H2A ubiquitin E3 ligase activity. Taken together, we suggest an integral role for EED as an epigenetic exchange factor coordinating the activities of PRC1 and 2. Polycomb group (PcG) proteins play a vital role in establishing and maintaining gene expression patterns during cellular differentiation and development [1] , [2] . PcG proteins function as multimeric, chromatin-associated protein complexes and are responsible for the repression of target genes [1] , [2] . The two major polycomb repressive complexes in mammals namely, PRC2 and PRC1, regulate the epigenome through methylation of histone H3K27 (refs 3 , 4 , 5 ), as well as the mono-ubiquitination of histone H2AK119, respectively [6] , [7] , [8] . The major components of human PRC2 include the histone methyltransferase, enhancer of Zeste homologue 2 (EZH2), and its known binding partners, embryonic ectoderm development (EED) and suppressor of Zeste 12 (SUZ12) [3] , [4] , [5] , [9] . While the human PRC1 consists of B lymphoma Mo-MLV insertion region 1 (BMI1), RING1A (also known as RING1) and RING1B (also known as RING2 or RNF2) [1] , [2] , [10] . Importantly, various components of both PRC1 and PRC2 have been shown to be elevated in a number of tumour types and play a critical role in neoplastic progression [11] , [12] , [13] , [14] , [15] . The leading hypothesis regarding the PRC2 and PRC1 interaction is that PRC2-mediated tri-methylation of H3K27 recruits PRC1 to genomic loci leading to chromatin condensation and epigenetic silencing of target genes [1] , [2] . While the evidence linking PRC1 and PRC2 is circumstantial, a physical or molecular link between these complexes has not been established. In this study, we make the unexpected observation that EED, previously considered a critical component of PRC2, is instead a shared component of PRC2 and PRC1 that functions to interchange these epigenetic complexes at sites of histone modification. This observation markedly enhances our understanding of how PRC2 and PRC1 coordinate epigenetic regulation and may have implications in therapeutically targeting these master regulators of transcription. EED binds directly to PRC1 proteins Relatively recently, JARID2 (jumonji homologue) has been reported to interact with PRC2 and regulate its function [16] , [17] , [18] , [19] , [20] . To identify novel PRC2 components or regulators we performed tandem mass spectrometric (MS) analysis individually of endogenous EZH2, EED and SUZ12 in VCaP prostate cancer cells ( Supplementary Fig. 1 ). 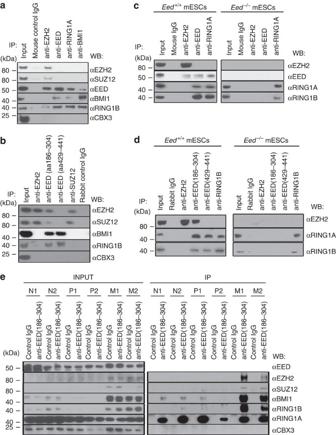Figure 1: PRC2 protein EED interacts with PRC1 proteins. (a) Immunoprecipitation of DU145 cell lysates with the indicated mouse monoclonal antibodies anti-EZH2, anti-EED (Millipore, cat# 05–1320), anti-SUZ12, anti-BMI1, anti-RING1A and control IgG was followed by immunoblot analysis. Anti-CBX3 was used as a negative control. Representative experiment from at least three independent analyses is shown for this and subsequent analyses. (b) Immunoprecipitation of DU145 lysates with the indicated rabbit polyclonal antibodies anti-EZH2, anti-EED (aa186–304) (Santa Cruz, cat# sc-28701), anti-EED (aa429–441) (Millipore, cat# 09–774), anti-SUZ12 and control IgG was followed by immunoblot analysis. (c) Immunoprecipitation ofEed+/+andEed−/−mESCs cell lysates with the indicated mouse monoclonal antibodies anti-EZH2, anti-EED (Millipore, cat# 05–1320), anti-RING1A and control IgG was followed by immunoblot analysis. Representative experiment from at least three independent analyses is shown for this and subsequent analyses. (d) Immunoprecipitation ofEed+/+andEed−/−mESCs cell lysates with the indicated rabbit polyclonal antibodies anti-EZH2, anti-EED (aa186–304) (Santa Cruz, cat# sc-28701), anti-EED (aa429–441) (Millipore, cat# 09–774), anti-RING1B and control IgG was followed by immunoblot analysis. (e) Immublot analysis of endogenous EED pull down (rabbit control IgG or anti-EED aa186–304) using lysates from normal prostate (N1 and N2), localized prostate cancer (P1 and P2) and metastatic prostate cancer tissues (M1 and M2). As expected, antibodies against EZH2 or SUZ12 co-immunoprecipitated known interactors of PRC2 such as EED, AEBP2, RBBP4 and RBBP7 ( Supplementary Table 1 and Supplementary Data 1 and 2 ). However, to our surprise, pull down of EED using a monoclonal antibody (Millipore Cat# 05–1320) and a polyclonal antibody (Millipore Cat# 09–774) failed to co-immunoprecipitate components of PRC2, and instead pulled down the PRC1 complex including core components such as BMI1 and RING1B ( Supplementary Fig. 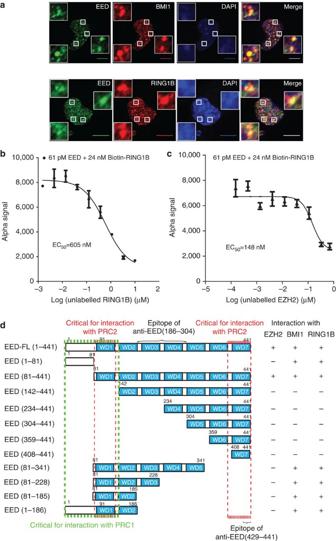Figure 2: N terminus of EED directly interacts with PRC1 proteins. (a) Confocal immunofluorescence analysis of EED (green) and BMI1 (red, top panels) or RING1B (red, bottom panels) in DU145 cells. DNA was counterstained with DAPI (blue). Insets are the magnified areas of co-localization. Scale bar, 10 μm. IF antibodies: mouse monoclonal anti-EED (Millipore, cat# 05–1320), anti-BMI1 and anti-RING1B antibodies. (b,c) Inhibition of biotin-RING1B and EED binding by unlabelled RING1B (b) or EZH2 (c) in the AlphaScreen assay. The EC50values of untagged RING1B and EZH2 were 605 nM and 148 nM, respectively. Assays were repeated five times in duplicate. All error bars represent ±s.e.m. (d) Schematic domain structures and interaction analysis of EED and EED deletion mutants. 2 and Supplementary Data 3 ), similar to the MS results using anti-RING1B or anti-BMI1 antibodies ( Supplementary Table 2 , Supplementary Data 4 and 5 ). To validate these surprising MS results, we performed IP-MS with these distinct anti-EED antibodies in Eed +/+ and Eed −/− mouse embryonic stem cells (mESCs) [21] and Eed +/+ mouse extraembryonic endoderm stem cells (XEN) ( Supplementary Fig. 1 ). Both anti-EED antibodies pulled down EED and PRC1 proteins BMI1 and RING1B, but not other PRC2 proteins in XEN and Eed +/+ mESCs, and importantly anti-EED antibodies did not pull down any PRC1 or PRC2 proteins from Eed −/− mESCs, indicating the specificity of these anti-EED antibodies ( Supplementary Fig. 3 , Supplementary Data 6 and 7 ). We further confirmed the presence of these protein–protein interactions in an additional prostate cancer cell line DU145 by immunoprecipitation followed by western blot analysis ( Fig. 1a ). Reciprocal immunoprecipitation of PRC1 components BMI1 or RING1A pulled down EED but not EZH2 or SUZ12 ( Fig. 1a and Supplementary Fig. 4 ). Importantly, the interactions were unaffected upon increasing the stringency of IP ( Supplementary Fig. 5 ) or washing conditions ( Supplementary Fig. 6 ), and EED still pulled down PRC1 proteins regardless of the buffer conditions tested. To further investigate this enigmatic result, we employed two distinct rabbit polyclonal antibodies against amino acids 186–304 (aa186–304) or 429–441 (aa429–441) of EED, respectively. Interestingly, anti-EED (aa186–304) pulled down both PRC2 components (that is, EZH2 and SUZ12) and PRC1 components (BMI1 and RING1B), while anti-EED (aa429–441) pulled down only PRC1 components in DU145 ( Fig. 1b ), VCaP and LNCaP ( Supplementary Fig. 4 ) cells. This suggested that anti-EED (aa429–441) masks an epitope at the extreme C terminus of EED that is required for interaction with PRC2 but not PRC1. Figure 1: PRC2 protein EED interacts with PRC1 proteins. ( a ) Immunoprecipitation of DU145 cell lysates with the indicated mouse monoclonal antibodies anti-EZH2, anti-EED (Millipore, cat# 05–1320), anti-SUZ12, anti-BMI1, anti-RING1A and control IgG was followed by immunoblot analysis. Anti-CBX3 was used as a negative control. Representative experiment from at least three independent analyses is shown for this and subsequent analyses. ( b ) Immunoprecipitation of DU145 lysates with the indicated rabbit polyclonal antibodies anti-EZH2, anti-EED (aa186–304) (Santa Cruz, cat# sc-28701), anti-EED (aa429–441) (Millipore, cat# 09–774), anti-SUZ12 and control IgG was followed by immunoblot analysis. ( c ) Immunoprecipitation of Eed +/+ and Eed −/− mESCs cell lysates with the indicated mouse monoclonal antibodies anti-EZH2, anti-EED (Millipore, cat# 05–1320), anti-RING1A and control IgG was followed by immunoblot analysis. Representative experiment from at least three independent analyses is shown for this and subsequent analyses. ( d ) Immunoprecipitation of Eed +/+ and Eed −/− mESCs cell lysates with the indicated rabbit polyclonal antibodies anti-EZH2, anti-EED (aa186–304) (Santa Cruz, cat# sc-28701), anti-EED (aa429–441) (Millipore, cat# 09–774), anti-RING1B and control IgG was followed by immunoblot analysis. ( e ) Immublot analysis of endogenous EED pull down (rabbit control IgG or anti-EED aa186–304) using lysates from normal prostate (N1 and N2), localized prostate cancer (P1 and P2) and metastatic prostate cancer tissues (M1 and M2). Full size image To further substantiate our results, we performed size-exclusion chromatography of nuclear extracts from VCaP, LNCaP and DU145 cells ( Supplementary Fig. 7a –c) and performed IP of EED and BMI1 from pools of different fractions as indicated. As shown in Supplementary Fig. 7d , EED pulled down BMI1, RING1A and RING1B in EED-positive fractions. To further confirm these findings, we performed IP immunoblot analysis in Eed +/+ and Eed −/− mESCs [21] ( Fig. 1c,d ), Eed +/+ XEN ( Supplementary Fig. 8a ) and BT549 breast cancer cell lysates ( Supplementary Fig. 8b ). While EED peptides were undetected in our MS of BMI1 or RING1B in VCaP cells, IP-western analyses in DU145, mESCs, XEN and BT549 using anti-BMI1 or RING1A antibodies clearly demonstrated the presence of EED protein ( Fig. 1a,c and Supplementary Fig. 8 ). Taken together, these data confirmed that the interaction between EED and PRC1 exists in both normal stem cells and cancer cells. A search of previously published EED MS data [5] , [17] , [18] revealed that most studies used an N-terminal FLAG-tagged EED construct and immunoprecipitated with anti-FLAG antibodies. To explore possible reasons as to why previous studies failed to detect the EED–PRC1 interaction, we constructed N-terminal and C-terminal FLAG-tagged versions of EED and overexpressed the proteins in HEK293 cells. Intriguingly, while N-terminal FLAG-tagged EED exclusively pulled down only PRC2 proteins, the C-terminal FLAG-tagged EED pulled down both PRC2 and PRC1 proteins ( Supplementary Fig. 9 ), suggesting that binding of anti-FLAG antibodies at the EED N terminus may hinder the EED–PRC1 interaction. In addition, ectopic overexpression of Halo-tagged full-length EED in HEK293 cells pulled down both PRC1 and PRC2, while ectopic expression of EED (aa1–186) bound only PRC1 ( Supplementary Fig. 10 ). When we overexpressed full-length EED along with N-terminal- and C-terminal-truncated mutations in Eed −/− mESCs, full-length EED was able to pull down both PRC2 and PRC1. By contrast, both truncated EED proteins could not bind PRC2 while the C terminal EED truncation mutant containing amino acids 1–186 maintained its interaction with PRC1 proteins ( Supplementary Fig. 11 ). IP-western blot analysis with or without ethidium bromide (EtBr) showed that the EED–EZH2 and EED–BMI1/RING1B interactions are not DNA dependent ( Supplementary Fig. 12 ). In addition to the various cell lines, we also observed the EED–PRC1 interaction in human prostate tissues including benign prostate, localized prostate cancer and metastatic prostate cancer samples ( Fig. 1e ). The above results further establish that EED is indeed a bona fide component of PRC1 in vivo . To assess potential co-localization of EED and PRC1 in cells, we performed immunofluorescence (IF) analysis using antibodies against EED, BMI1, RING1B, EZH2 and SUZ12 in DU145 cells ( Fig. 2a and Supplementary Fig. 13 ) and LNCaP cells ( Supplementary Fig. 14 ). Consistent with the immunoprecipitation studies, 66.6% and 60.3% of EED overlapped BMI1 and RING1B, respectively, by quantitative IF analysis (see Methods for details). Figure 2: N terminus of EED directly interacts with PRC1 proteins. ( a ) Confocal immunofluorescence analysis of EED (green) and BMI1 (red, top panels) or RING1B (red, bottom panels) in DU145 cells. DNA was counterstained with DAPI (blue). Insets are the magnified areas of co-localization. Scale bar, 10 μm. IF antibodies: mouse monoclonal anti-EED (Millipore, cat# 05–1320), anti-BMI1 and anti-RING1B antibodies. ( b , c ) Inhibition of biotin-RING1B and EED binding by unlabelled RING1B ( b ) or EZH2 ( c ) in the AlphaScreen assay. The EC 50 values of untagged RING1B and EZH2 were 605 nM and 148 nM, respectively. Assays were repeated five times in duplicate. All error bars represent ±s.e.m. ( d ) Schematic domain structures and interaction analysis of EED and EED deletion mutants. Full size image To determine whether EED and PRC1 components interact directly and assess their binding affinity, we developed an AlphaScreen assay using purified full-length EED and RING1B proteins ( Fig. 2b and Supplementary Fig. 15a ). As shown in Fig. 2b , purified full-length EED directly interacts with full-length RING1B with an EC 50 605 nM, comparable to the previously reported binding affinity of 380 nM between EZH2 (aa39–68) and full-length EED [22] . While the full-length EZH2 could competitively bind to EED and displace RING1B ( Fig. 2c ), this effect was not observed with the negative control full-length KRAS ( Supplementary Fig. 15b ). To define the domains of EED required for its interaction with PRC1 and PRC2, we took the advantage of a cell-free in vitro wheat germ translation system, designed a series of human EED isoforms ( Supplementary Fig. 16a ) and deletion constructs ( Fig. 2d ), and characterized the epitopes for all three anti-EED antibodies used in this study ( Supplementary Fig. 16b and 16c ). As shown, the monoclonal anti-EED antibody (Millipore, cat# 05–1320) and polyclonal anti-EED antibody (Millipore, Cat# 09–774) do not recognize human EED isoform C (missing aa 401–441, the 7th WD40 motif). The polyclonal anti-EED antibody (Santa Cruz, Cat# sc-28701) recognized all human isoforms and aa186–304 sequence is the immunoreactive epitope. By biochemical interaction studies ( Supplementary Fig. 17 ), we found that the N-terminal amino acids 1–186 of EED are critical for binding to PRC1 while aa81–141 and aa429–441 are critical for PRC2 binding ( Supplementary Fig. 17 ). The anti-EED antibodies that recognize the 7th WD40 motif appear to block an interaction site that is required for PRC2 binding [22] , [23] . A summary of this interaction analysis is provided in Fig. 2d . EED–EZH2 interaction is disrupted by EED C-terminal antibodies Next, we explored whether the EED antibody (aa429–441) may block PRC2 function since it appears to interfere with EZH2 binding. Increasing concentrations of the anti-EED (aa429–441) antibody disrupted the interaction between EZH2 and EED in vitro which was not the case for an anti-EED (aa186–304) antibody or a control IgG ( Fig. 3a ). We next examined whether the anti-EED (aa429–441) antibody could block the function of PRC2. To test this, we performed an in vitro H3K27 tri-methylation assay using purified recombinant PRC2 complex, recombinant unmodified histone H3 ( Fig. 3b ) and nucleosomes ( Fig. 3c ) as substrates with anti-EED (aa429–441), anti-EED (aa186–304) and control IgG antibodies. As previously reported [3] , [4] , [5] , [9] , PRC2 requires EED to methylate histone H3K27 and this was the case in the assays we carried out ( Fig. 3b,c ). Interestingly, addition of the anti-EED (aa429–441) antibody attenuated PRC2 activity in a dose-dependent manner, while anti-EED (aa186–304) antibody and control IgG did not ( Fig. 3b,c ), confirming that the interaction between EED and EZH2 is critical for PRC2 activities. Therefore, as the anti-EED (aa429–441) antibody is a potent inhibitor of PRC2 function in vitro , small molecules targeting this interaction interface may block PRC2 activity with a mechanism of action distinct from inhibition of the enzymatic SET domain of EZH2 (refs 24 , 25 , 26 ). 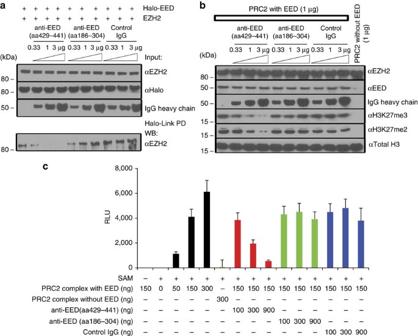Figure 3: Anti-EED (aa429–441) antibody disrupts PRC2 and attenuates its histone methyltransferase activity. (a) Anti-EED (aa429–441) antibody inhibits the EED–EZH2 interaction. Halo-tagged full-length EED protein was incubated with EZH2 in the presence of different amounts of control IgG, anti-EED (aa429–441) and anti-EED (aa186–304) antibodies. Halo-Link PD (pull down) followed by immunoblot analysis is shown. (b) Anti-EED (aa429–441) antibody inhibits PRC2-mediated methylation of histone H3in vitro. Indicated amounts of purified PRC2, control IgG, anti-EED (aa429–441) and anti-EED (aa186–304) antibodies were incubated with recombinant histone H3 with unmethylated H3K27 for 2 h. Immunoblot analyses with anti-H3K27me3 and anti-H3K27me2 antibodies were then performed. (c) Anti-EED (aa429–441) antibody inhibits PRC2-mediated methylation of nucleosomesin vitro. Indicated amounts of purified PRC2, control IgG, anti-EED (aa429–441) and anti-EED (aa186–304) antibodies were incubated with nucleosomes containing unmethylated H3K27. ELISA with anti-H3K27me3 antibody was then performed to measure PRC2 histone methyltransferase activity. Assays were repeated three times in triplicate. All error bars represent ±s.e.m. Figure 3: Anti-EED (aa429–441) antibody disrupts PRC2 and attenuates its histone methyltransferase activity. ( a ) Anti-EED (aa429–441) antibody inhibits the EED–EZH2 interaction. Halo-tagged full-length EED protein was incubated with EZH2 in the presence of different amounts of control IgG, anti-EED (aa429–441) and anti-EED (aa186–304) antibodies. Halo-Link PD (pull down) followed by immunoblot analysis is shown. ( b ) Anti-EED (aa429–441) antibody inhibits PRC2-mediated methylation of histone H3 in vitro . Indicated amounts of purified PRC2, control IgG, anti-EED (aa429–441) and anti-EED (aa186–304) antibodies were incubated with recombinant histone H3 with unmethylated H3K27 for 2 h. Immunoblot analyses with anti-H3K27me3 and anti-H3K27me2 antibodies were then performed. ( c ) Anti-EED (aa429–441) antibody inhibits PRC2-mediated methylation of nucleosomes in vitro . Indicated amounts of purified PRC2, control IgG, anti-EED (aa429–441) and anti-EED (aa186–304) antibodies were incubated with nucleosomes containing unmethylated H3K27. ELISA with anti-H3K27me3 antibody was then performed to measure PRC2 histone methyltransferase activity. Assays were repeated three times in triplicate. All error bars represent ±s.e.m. Full size image PRC1 members compete with EZH2 for EED To investigate whether PRC1 components BMI1 or RING1B could compete with EZH2 for EED binding, we carried out an in vitro competition experiment using the in vitro translated proteins. Interestingly, increasing concentrations of BMI1 or RING1B competitively sequestered EED protein and prevented its interaction with EZH2 ( Fig. 4a ). Similarly, increasing concentrations of EZH2 competitively sequestered EED protein and prevented its interaction with BMI1 ( Supplementary Fig. 18 ). Next, we assessed whether increasing concentrations of PRC1 components BMI1 or RING1B could inhibit the enzymatic function of PRC2. Using recombinant unmodified histone H3 or purified nucleosomes, increasing the levels of BMI1 or RING1B abrogated PRC2 enzymatic activity ( Fig. 4b,c ). Both di- and tri-methylation of H3K27 were inhibited by PRC1 ( Fig. 4b ). 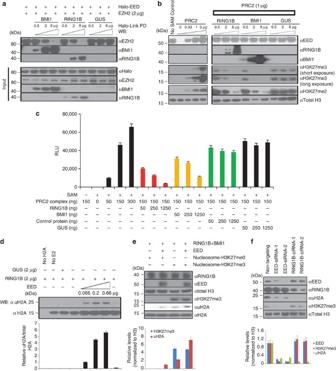Figure 4: The EED–PRC1 interaction alters PRC2 histone methyltransferase and PRC1 histone ubiquitin E3 ligase activities. (a) PRC1 proteins disassociate EED–EZH2 complexes. EZH2 protein was incubated with halo-tagged EED in the presence of different amounts of BMI1, RING1B or GUS proteins. Halo-Link PD followed by immunoblot analysis was performed. (b) BMI1 and RING1B inhibit PRC2-mediated methylation of histone H3in vitro. Indicated amounts of purified PRC2, RING1B, BMI1 and GUS were incubated with recombinant histone H3 with unmethylated H3K27 for 2 h. Immunoblot analyses with anti-H3K27me3 and anti-H3K27me2 antibodies were then performed. (c) BMI1 and RING1B inhibit PRC2-mediated methylation of nucleosomesin vitro. Indicated amounts of purified recombinant PRC2, RING1B, BMI1 and GUS proteins were incubated with nucleosomes containing unmethylated H3K27. ELISA with anti-H3K27me3 antibody was then performed. Assays were repeated thrice in triplicates. All error bars represent ±s.e.m. (d) EED enhances RING1B-mediated ubiquitination of histone H2Ain vitro. Indicated amounts of purified EED, RING1B, BMI1 and GUS were incubated with recombinant histone H2A for 1 h. Immunoblot analyses with anti-uH2A antibody were then performed to measure histone H2A ubiquitin E3 ligase activity. Assays were independently repeated three times. Normalized band intensity by densitometry from the three independent assays is represented as bar graphs below the immunoblot. Error bars represent ±s.e.m. (e) EED enhances PRC1-mediated ubiquitination of nucleosome H2Ain vitro. Purified EED, RING1B, BMI1 and GUS were incubated with reconstituted mono-nucleosomes with un- or tri-methylated H3K27. Immunoblot analyses with anti-uH2A antibody were then performed to measure histone H2A ubiquitin E3 ligase activity. Normalized band intensity by densitometry from three independent assays is represented as bar graphs blow the immunoblot. Error bars represent ±s.e.m. (f) Knockdown of EED and RING1B altered H3K27me3 and uH2A levels in cells. EED- and RING1B-specific siRNA duplexes and non-targeting control were transfected into DU145 cells. Expression levels of indicated proteins were assessed by immunoblot analysis. Normalized band intensity by densitometry from three independent assays is represented as bar graphs blow the immunoblot. All error bars represent ±s.e.m. Figure 4: The EED–PRC1 interaction alters PRC2 histone methyltransferase and PRC1 histone ubiquitin E3 ligase activities. ( a ) PRC1 proteins disassociate EED–EZH2 complexes. EZH2 protein was incubated with halo-tagged EED in the presence of different amounts of BMI1, RING1B or GUS proteins. Halo-Link PD followed by immunoblot analysis was performed. ( b ) BMI1 and RING1B inhibit PRC2-mediated methylation of histone H3 in vitro . Indicated amounts of purified PRC2, RING1B, BMI1 and GUS were incubated with recombinant histone H3 with unmethylated H3K27 for 2 h. Immunoblot analyses with anti-H3K27me3 and anti-H3K27me2 antibodies were then performed. ( c ) BMI1 and RING1B inhibit PRC2-mediated methylation of nucleosomes in vitro . Indicated amounts of purified recombinant PRC2, RING1B, BMI1 and GUS proteins were incubated with nucleosomes containing unmethylated H3K27. ELISA with anti-H3K27me3 antibody was then performed. Assays were repeated thrice in triplicates. All error bars represent ±s.e.m. ( d ) EED enhances RING1B-mediated ubiquitination of histone H2A in vitro . Indicated amounts of purified EED, RING1B, BMI1 and GUS were incubated with recombinant histone H2A for 1 h. Immunoblot analyses with anti-uH2A antibody were then performed to measure histone H2A ubiquitin E3 ligase activity. Assays were independently repeated three times. Normalized band intensity by densitometry from the three independent assays is represented as bar graphs below the immunoblot. Error bars represent ±s.e.m. ( e ) EED enhances PRC1-mediated ubiquitination of nucleosome H2A in vitro . Purified EED, RING1B, BMI1 and GUS were incubated with reconstituted mono-nucleosomes with un- or tri-methylated H3K27. Immunoblot analyses with anti-uH2A antibody were then performed to measure histone H2A ubiquitin E3 ligase activity. Normalized band intensity by densitometry from three independent assays is represented as bar graphs blow the immunoblot. Error bars represent ±s.e.m. ( f ) Knockdown of EED and RING1B altered H3K27me3 and uH2A levels in cells. EED- and RING1B-specific siRNA duplexes and non-targeting control were transfected into DU145 cells. Expression levels of indicated proteins were assessed by immunoblot analysis. Normalized band intensity by densitometry from three independent assays is represented as bar graphs blow the immunoblot. All error bars represent ±s.e.m. Full size image We next explored whether EED enhances the functional activities of PRC1. Employing an in vitro H2A ubiquitination assay, we assessed whether EED affects the E3 ubiquitin ligase activity of RING1B. Similar to BMI1 ( Supplementary Fig. 19 ) [6] , EED enhanced RING1B-mediated ubiquitination of histone H2A in a dose-dependent manner ( Fig. 4d ). Using reconstituted mono-nucleosomes as substrates ( Supplementary Fig. 20 ), the RING1B-BMI1 complex without EED had minimal activity on the ubiquitination of H2A in nucleosomes with unmethylated H3K27, but, in the presence of EED, the PRC1 complex strongly ubiquitinated H2A ( Fig. 4e ). Interestingly, while the RING1B–BMI1 complex could ubiquitinate H2A of the nucleosomes with H3K27me3, EED markedly enhanced this activity ( Fig. 4e ), indicating that EED is critical for recruiting PRC1 to H3K27me3 marked loci to perform its function. To investigate the role of EED in PRC1 function in vivo , we carried out knockdown studies in cell lines. As expected, knockdown of RING1B led to global decreases in ubiquitinated H2A but not H3K27me3 ( Fig. 4f ). More importantly, knockdown of EED attenuated global levels of both ubiquitinated H2A and H3K27me3 ( Fig. 4f ), supporting the critical role of EED in both PRC1 and PRC2 function. EED recruits PRC1 to PcG target loci To understand the long-term effects of EED dysregulation, we stably knocked down EED by two different EED-specific shRNA constructs in DU145 and LNCaP cells ( Supplementary Fig. 21a ). Similar to EZH2 stable knockdown, decreased EED inhibited proliferation ( Supplementary Fig. 21b,c ) and invasiveness ( Supplementary Fig. 21d ) of DU145 and LNCaP cells. Furthermore, murine xenograft models showed that stably knocking down EED significantly repressed tumour formation and growth ( Supplementary Fig. 21e ). To examine the role of EED in the localization of PRC1, PRC2 and associated histone marks, we carried out a series of ChIP-qPCR experiments across a set of classic PRC1 and PRC2 target genes employing the most efficient EED knockdown cell line from above (EED-sh3 described in Supplementary Fig. 21 ) and a matched vector control cell line. Recruitment of PRC1, PRC2, H3K27me3 and ubiquitinated H2A were all markedly reduced in PRC2 targets ADRB2 , MYT and CNR [17] , [18] and PRC1 target genes p16INK4A , p19 and HOXC13 (refs 6 , 11 , 27 ) when EED was knocked down ( Fig. 5a ). This was not the case in control genes NUP214 or KIAA0066 . Further, ChIP-qPCR experiments using EZH2 ( Supplementary Fig. 21a ), SUZ12 ( Supplementary Fig. 22a ) and RING1B [11] stable knockdown cell lines showed that knockdown of EZH2 and SUZ12 reduced EED protein levels ( Supplementary Figs 21a and 22a ) [28] , [29] , resulting in decreased recruitment of EED, EZH2, SUZ12, RING1B, H3K27me3 and uH2A in PRC2 and PRC1 target genes ( Supplementary Fig. 22b ). However, knockdown of RING1B merely decreased occupancy of RING1B, not PRC2 proteins, at PcG target gene promoters ( Supplementary Fig. 22b ). To extend this on a genome-wide scale, we performed EED, uH2A, EZH2, H3K27me3, BMI1, RING1A and RING1B ChIP-Sequencing (ChIP-Seq) using the same mouse monoclonal anti-EED antibody used for MS (which only pulls down PRC1 and not PRC2), anti-EZH2, anti-H3K27me3, anti-BMI1, anti-RING1A, anti-RING1B and two different (one monoclonal and one polyclonal) anti-uH2A antibodies. WNT1 , WNT8B and the HOXA cluster are examples of known PRC1 genomic target regions ( Supplementary Fig. 23a ). A total of 82.3% (3096/3764) EED occupied genes exhibited ubiquitination of H2A ( Fig. 5b ), which is consistent with previously reported genome-wide analyses of PRC2 and PRC1 targets [30] , [31] , [32] , [33] , [34] . Knockdown of EED markedly reduced the ubiquitination of H2A, BMI1, RING1A, RING1B and H3K27me3, as well as EED occupancy around the transcriptional start sites (TSSs) ( Fig. 5c and Supplementary Fig. 23b ). In addition, knockdown of EED decreased the number of uH2A-modified genes ( Fig. 5d ). Overall, the occupancy of uH2A modification, BMI1, RING1A, RING1B and EED on promoter regions was remarkably reduced by knockdown of EED ( Fig. 5e and Supplementary Fig. 23c ). As expected, EZH2 occupancy on promoter regions was decreased by knockdown of EED ( Supplementary Fig. 23d ). The shared or unique PRC2 (EZH2 occupied genes) and PRC1 (uH2A occupied genes) target genes were listed in the Supplementary Data 8 . Examples of EED–PRC1 unique target loci were shown in Supplementary Fig. 23e . Because the functions of PRC1 and PRC2 complexes are highly interconnected, the functions of EED in the PRC1 complex could not be completely distinguished from EED in the PRC2 complex. To further corroborate our results directly linking EED and PRC1, we examined a published data set in which RING1B ChIP-Seq was carried out in Eed +/+ or Eed −/− mouse embryonic stem cells (mESCs) [35] . Overall, the occupancies of RING1B on promoter regions in Eed −/− mESCs was significantly diminished relative to that of Eed +/+ mESCs ( Fig. 6a–c ). Taken together, these data suggest that EED is critical for PRC1 binding to target loci. 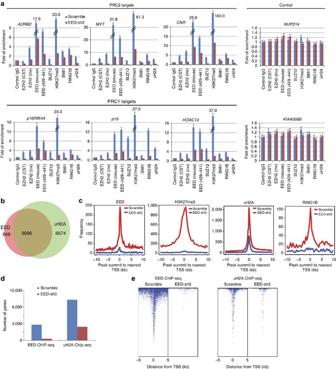Figure 5: EED is critical for PRC1 recruitment to target genes. (a) ChIP-qPCR analysis of indicated proteins at PRC2 target genesADRB2,MYT1andCNRand PRC1 target genesp16INK4A/CDKN2A,p19/CDKN2DandHOXC13.NUP214andKIAA0066were used as negative controls. Antibodies used for ChIP: mouse control IgG, rabbit control IgG, anti-EZH2 (CST) (Cell Signaling, cat# 5246), anti-EZH2 (Inv) (Invitrogen, cat# 49–1043), anti-EED (Millipore, cat# 05–1320), anti-EED (aa429–441) (Millipore, cat# 09–774), anti-SUZ12, anti-BMI1, anti-RING1B, anti-H3K27me3 and anti-uH2A. ChIP assays were biologically repeated twice, and qPCR analyses were done in triplicate. All error bars represent ±s.e.m. (b) Venn diagrams show that 82.3% of EED bound genes in DU145 cells are also enriched with uH2A. (c) Knockdown of EED attenuates the occupancy of EED, uH2A, H3K27me3 and RING1B at PcG target promoters. Genome-wide patterns of uH2A modification, H3K27me3, EED and RING1B in DU145 scramble control cells (red) and DU145 EED-sh3 cells (blue) are noted at all annotated gene promoters. (d) Bar graph of genes with EED occupancy (left panel) and uH2A (right panel) modification in scramble or EED-sh3 cells. (e) Heatmap representation of genomic regions with binding profiles of EED (left panel) and uH2A (right panel) in DU145 scramble or EED-sh3 cells 5 kb flanking the transcriptional start site of genes. Figure 5: EED is critical for PRC1 recruitment to target genes. ( a ) ChIP-qPCR analysis of indicated proteins at PRC2 target genes ADRB2 , MYT1 and CNR and PRC1 target genes p16INK4A/CDKN2A , p19/CDKN2D and HOXC13 . NUP214 and KIAA0066 were used as negative controls. Antibodies used for ChIP: mouse control IgG, rabbit control IgG, anti-EZH2 (CST) (Cell Signaling, cat# 5246), anti-EZH2 (Inv) (Invitrogen, cat# 49–1043), anti-EED (Millipore, cat# 05–1320), anti-EED (aa429–441) (Millipore, cat# 09–774), anti-SUZ12, anti-BMI1, anti-RING1B, anti-H3K27me3 and anti-uH2A. ChIP assays were biologically repeated twice, and qPCR analyses were done in triplicate. All error bars represent ±s.e.m. ( b ) Venn diagrams show that 82.3% of EED bound genes in DU145 cells are also enriched with uH2A. ( c ) Knockdown of EED attenuates the occupancy of EED, uH2A, H3K27me3 and RING1B at PcG target promoters. Genome-wide patterns of uH2A modification, H3K27me3, EED and RING1B in DU145 scramble control cells (red) and DU145 EED-sh3 cells (blue) are noted at all annotated gene promoters. ( d ) Bar graph of genes with EED occupancy (left panel) and uH2A (right panel) modification in scramble or EED-sh3 cells. ( e ) Heatmap representation of genomic regions with binding profiles of EED (left panel) and uH2A (right panel) in DU145 scramble or EED-sh3 cells 5 kb flanking the transcriptional start site of genes. 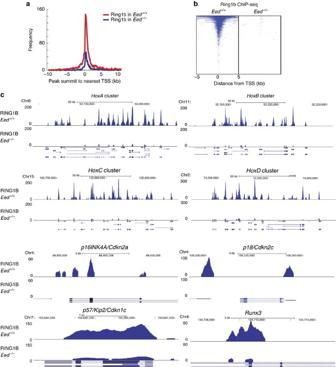Figure 6: EED Knockdown abolishes RING1B occupancy on target genes. (a) EED is crucial for RING1B binding to PcG target promoters. Genome-wide occupancies of RING1B inEed+/+mESCs (red) andEed−/−mESCs (blue) are noted at all annotated gene promoters. Data from Tavareset al.35was utilized. (b) Heatmap representation of genomic regions with binding profiles of RING1B inEed+/+andEed−/−mESCs at genes 5 kb flanking TSSs. (c) Differential RING1B binding betweenEed+/+mESCs andEed−/−mESCs samples in various target genomic regions are shown. Full size image Figure 6: EED Knockdown abolishes RING1B occupancy on target genes. ( a ) EED is crucial for RING1B binding to PcG target promoters. Genome-wide occupancies of RING1B in Eed +/+ mESCs (red) and Eed −/− mESCs (blue) are noted at all annotated gene promoters. Data from Tavares et al. [35] was utilized. ( b ) Heatmap representation of genomic regions with binding profiles of RING1B in Eed +/+ and Eed −/− mESCs at genes 5 kb flanking TSSs. ( c ) Differential RING1B binding between Eed +/+ mESCs and Eed −/− mESCs samples in various target genomic regions are shown. Full size image Significant advances have been made towards understanding the role of PRCs in regulating heritable gene silencing during differentiation, development and neoplastic progression [1] , [2] , [24] , [36] . The prevailing dogma suggests that EED functions as the H3K27me3 binding subunit of PRC2 and, through this interaction, enhances the enzymatic activity of PRC2 forming a positive feedback loop [37] . It is also thought that PRC1 functions downstream of PRC2, binding to H3K27me3, and subsequently enacting H2AK119 ubiquitination to maintain gene silencing [1] , [8] . In this study, we carried out mass spectrometric analysis of endogenous PRC complexes in cancer and normal stem cell lines. Incidentally, we employed an antibody to immunoprecipitate endogenous EED, which interacted within a site in EED that prevented interaction with PRC2. Quite surprisingly, this EED immunoprecipitate revealed proteins in the PRC1 complex including BMI1, RING1A, RING1B, CBXs and PHCs. Antibodies that block the EED interaction with PRC2 inhibit PRC2 activity while maintaining interaction with PRC1. Incubating PRC1 components BMI1 or RING1B competitively displaced the interaction of EED with PRC2. Similar to the known function of EED in enhancing PRC2 activity [4] , [9] , in this study, although EED’s function could not be dissected from PRC2 function, we demonstrated that EED also enhances PRC1 activity in terms of ubiquitination of H2AK119. Recent studies suggest that there are at least two forms of PRC1, containing either CBX components or RYBP protein [35] , [38] , [39] . Several groups have reported that, in embryonic stem cells, the histone demethylase KDM2B can interact and recruit RYBP-PRC1 complex containing PCGF1, a homologue of BMI1 (PCGF4), to CpG islands [40] , [41] , [42] and is essential for H2A mono-ubiquitination [42] . Our MS analysis carried out in VCaP prostate cancer cells suggests that the interaction of KDM2B and RING1B exists in prostate cancer as well ( Supplementary Data 4 ). Importantly, our study demonstrates that EED is part of the CBX-containing PRC1 complexes as our EED pull down proteins are almost identical to members of RING1B-BMI1 (PCGF4) and RING1B-MEL18 (PCGF2) complexes ( Supplementary Data 3 ) [39] . In addition, while BMI1, RING1B and several CBXs were detected at high frequency in the immunoprecipitates, RYBP, KDM2B, PCGF1, PCGF5 and PCGF6 were represented at a low frequency. This would potentially explain the residual ubiquitination activity of the RYBP–PRC1 complex in EED knockout mice [35] . As shown in our independent analysis and interpretation of their RING1B ChIP-Seq data ( Fig. 6a–c ), we demonstrate that global H2A ubiquitination at transcription start sites and proximal promoter regions of target genes is markedly attenuated, presumably caused by loss of EED–CBX-containing PRC1 in Eed −/− cells. The remaining H2A ubiquitination activity is likely mediated by the RYBP-containing PRC1, which functions independently of EED (that is, PRC2). The decreased global uH2A levels we observed in Eed −/− mESCs, in contrast to previous reports [35] , [43] , suggest that the ubiquitination of H2A might be accomplished by distinct PRC1 complexes. The previously demonstrated roles of PRC1–CBXs or PRC1–RYBP may explain these differences [35] . While a sequential activity of PRC2 and PRC1 in mediating gene silencing has been postulated [1] , [8] , the mechanism remained unclear. Here, we propose a model in which EED plays a central role interacting with H3K27 and enhancing H3K27me3 mediated by PRC2. Once H3K27 is trimethylated, EED recruits PRC1 leading to the displacement of PRC2 components, ubiquitination of H2AK119 and consequent gene silencing. Thus, EED may play a central role as an ‘epigenetic exchange factor’ orchestrating the sequential activities of PRC2 and PRC1 ( Fig. 7 ), a phenomenon that has remained unappreciated. 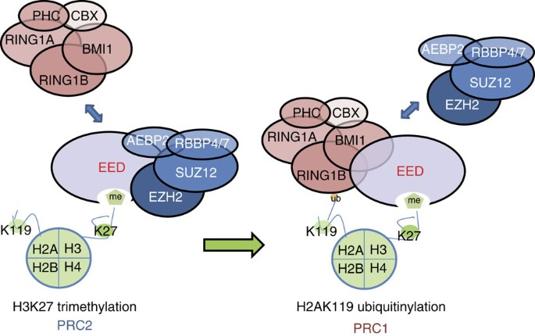Figure 7: The proposed model depicting a role for EED in orchestrating PRC2 and PRC1 function in epigenetic regulation. EED is critical for PRC2 to methylate histone H3 at lysine 27. Once H3K27 are methylated, EED directly recruits PRC1 to the tri-methylated H3K27 loci and enhances PRC1 ubiquitin E3 ligase activity. Figure 7: The proposed model depicting a role for EED in orchestrating PRC2 and PRC1 function in epigenetic regulation. EED is critical for PRC2 to methylate histone H3 at lysine 27. Once H3K27 are methylated, EED directly recruits PRC1 to the tri-methylated H3K27 loci and enhances PRC1 ubiquitin E3 ligase activity. Full size image Cell lines and reagents Prostate cancer cell lines namely, DU145, VCaP and LNCaP were grown in the 10% FBS (Invitrogen, Carlsbad, CA) containing MEM, DMEM with Glutamax and RPMI1640 (Invitrogen) respectively, under 5% CO 2 in a cell culture incubator. Lentiviruses were generated by the University of Michigan Vector Core. DU145 and LNCaP cells were infected with lentiviruses expressing either scramble shRNA or EZH2, EED specific shRNA duplexes containing GFP reporter. Stable cell lines were generated by selection with 1 μg ml −1 puromycin and monitored with GFP fluorescence. Eed −/− mouse stem cells were gift from Dr Terry Magnuson and grown in MEMalpha (Invitrogen) with 20% ES qualified FBS (ATCC, Manassas, VA), 1 mM sodium pyruvate (Invitrogen), 2 mM L -Glutamine (Invitrogen), 1X NEAA (Invitrogen), 100 μM β -Mercaptoethanol (Invitrogen), 1,000 units per ml LIF (Millipore, Billerica, MA). XEN cells were grown in MEMalpha with 20% ES qualified FBS, 1 mM Sodium Pyruvate, 2 mM L -Glutamine, 1 × NEAA (Invitrogen), 100 μM β-Mercaptoethanol. A list of antibodies with dilutions used for immunoprecipitation (IP), immunoblot, ChIP and Immuno-Fluorescence (IF) is presented in Supplementary Table 3 . Immunoprecipitation and mass spectrometry analysis VCaP cells were lysed in Triton X-100 lysis buffer (20 mM MOPS, pH 7.0, 2 mM EGTA, 5 mM EDTA, 30 mM sodium fluoride, 60 mM β-glycerophosphate, 20 mM sodium pyrophosphate, 1 mM sodium orthovanadate, 1% Triton X-100, 1 mM DTT, protease inhibitor cocktail (Roche, Indianapolis, IN, #14309200)). VCaP Cell lysates (0.5–1.0 mg), mouse embryonic stem cells (mESCs) and extraembryonic endoderm stem cells (XEN) nuclear extracts (2.5 mg) in RIPA buffer were pre-cleaned with protein A/G agarose beads (Santa Cruz, # sc-2003) by incubation for 1 h with rotating at 4 °C, followed by centrifugation at 2,000 r.p.m. for 3 min. Lysates were then incubated with respective antibodies and Dynabeads (Invitrogen) at 4 °C overnight before washing the lysate-bead precipitate (centrifugation at 2,000 r.p.m for 3 min) 4 times in Triton X-100 lysis buffer or RIPA buffer. Beads were then precipitated by centrifugation, resuspended in 25 μl of 2 × loading buffer and boiled at 85 °C for 5 min to separate the protein and beads. Eluted proteins were then alkylated by 15 mM iodoacetamide for 10 min. Samples were then analysed by SDS-PAGE western blot analysis as described below [44] . In parallel, IP eluate was resolved with SDS-PAGE and visualized with silver stain (PROTSIL-2, Sigma) or Coomassie blue stain. Each gel lane, experimental or control, was into several pieces for in-gel trypsin digestion in accordance with the manufacturer’s instructions. The samples were incubated with trypsin (1:20) enzyme:protein (w:w) overnight at 37 °C. Peptides were then extracted from the gel, lyophilized to dryness and stored at −80 °C until further analysis. Chromatography was performed on a nanoLC system (Proxeon). The peptides were loaded on C18 peptide trap and eluted onto C18 column (10 cm long, 75 um ID, 3 μm HALO resin (Michrom)) with a 1 h linear gradient of acetonitrile. The peptides were analysed by using a LTQ Velos Pro mass spectrometer operating in a data-dependent mode. Original spectrum files (.raw) were converted to MGF format using MSConverter. The resulting.xml files were interrogated by X!Tandem using human or mouse UniProt database supplied with a complete set of reverse sequences for false discovery rate (FDR) estimation.The search settings specified trypsin as the protease, maximum of two missed cleavage sites, precursor charge up to 4+, excluding singly charged species, 0.8 Dalton (Da) fragment ion tolerance and −1/+4 Da for precursor ion tolerance. For data presented in the Supplementary Data 3, 6 and 7 the resulting files were analysed by PeptideProphet [45] and ProteinProphet [46] , and the proteins were filtered at the probability of 0.95. For quantitation by spectral counting, the results from all experiments were compiled using Abacus software [47] for grouping of the related proteins, removing redundant hits and adjustment of the shared spectral counts. For data presented in the Supplementary Data 1, 2, 4 and 5 the following analysis procedure was employed. X!Tandem results were analysed by PeptideProphet and ProteinProphet. A tabulated listing of confidently identified proteins was filtered for statistical significance at a calucated false discovery rate of 5%; which correlated to a 60% Protein Probability and 95% PeptideProbability. This listing then was manually curated to remove all proteins found commonly as contaminants among affinity purification-mass spectrometry (AP-MS) experiments. The AP-MS contaminate listing was generated in-house exactly as described above representing a collated listing from five biological replicates of VCaP IgG bound Dynabeads. Interaction assays A total of 100 μl of cell-free reaction containing EZH2, BMI1 or RING1B proteins were incubated with Halo-tagged EED full-length or subdomain fusion proteins in PBS-T (0.1% Tween 20) overnight at 4 °C. In parallel, 10 μl of Halo-Link beads (Promega) were then blocked in BSA overnight at 4 °C. Following day, the beads were washed three times with PBS and mixed with Halo-EED:PcG mixture and incubated at RT for 1 h. Halo-Link beads were subjected to four washes with PBST, and the bound fraction was eluted in SDS loading buffer. Proteins were separated on SDS gel and blotted with indicated antibodies. GUS protein was used as a negative control. Immunofluorescence and co-localization analysis DU145 or LNCaP cells were fixed with 3.7% paraformaldehyde and then permeabilized with 0.1% (w/v) saponin (Sigma) for 15 min. Cells were co-incubated with primary antibodies against EED and BMI1 or EED and RING1B (1:100 dilution) for 12 h at 4 °C, followed by incubation with appropriate Alexa-Fluor-conjugated secondary antibodies (1:200 dilution) for 30 min at 37 °C. Cells were washed and mounted onto glass slides using Vectashield mounting medium (Vector Laboratories, Burlingame, CA) containing DAPI. Samples were analysed using a Nikon A1 laser-scanning confocal microscope equipped with a Plan-Apo × 63/1.4 numerical aperture oil lens objective. Acquired images were then analysed using ImageJ software (version 1.41). Co-localization was analysed in Image J software using JACoP plugin. Nuclei (15–20) were counted, and co-localization was measured using the Manders coefficient to evaluate the overlap in fluorescence. EED-RING1B alphascreen assay The AlphaScreen protocol from the manufacturer (PerkinElmer) was followed unless otherwise specified. Assay development and optimization was carried out in white 96-well half area plates, and all incubation steps were at room temperature (21 °C). In brief, biotinylated RING1B (biotin-RING1B) was captured by a streptavidin-coated donor bead, and EED is bound by an anti-EED mAb and AlphaLISA anti-mouse IgG acceptor bead. The binding of RING1B to EED brings the donor and acceptor beads in close proximity, enabling energy transfer between them, resulting in a chemiluminescence signal [48] . A competitor (that is, unlabelled RING1B protein) of the EED-RING1B interaction will disrupt the energy transfer between the donor and acceptor beads, resulting in a reduction of chemiluminescence signal. The signal amplification properties of the AlphaScreen method allow for the homogenous detection of protein–protein interactions with high sensitivity. To determine the binding affinity, 10 μl per well of 24 nM biotin-RING1B was incubated with 10 μl per well of 61pM EED for 1 h followed by the addition of 10 μg ml −1 streptavidin-coated donor beads and anti-EED mAb+AlphaLISA anti-mouse IgG acceptor beads at 10 μg ml −1 diluted in 25 mM HEPES, 150 mM NaCl, 0.1% BSA and 0.1% Tween. Unlabelled RING1B and EZH2 were titrated in as positive controls that displaced the binding of EED to biotin-RING1B. Unlabelled KRAS was used as negative control protein. The assay plate was incubated for 1 h with light shading before it was measured in a Tecan plate reader in AlphaScreen detection mode. Immunoblot analyses HEK293 cells, BT549, mESCs, XEN, prostate cancer cell lines DU145, LNCaP and VCaP, and prostate tissues were homogenized in NP-40 lysis buffer containing 50 mM Tris-HCl, pH 7.4, 1% Nonidet P-40 (Sigma, St Louis, MO) and complete protease inhibitor cocktail (Roche). Ten micrograms of each protein extract or IP elutes was boiled in sample buffer, separated by SDS-PAGE and transferred onto Polyvinylidene Difluoride membrane (GE Healthcare, Piscataway, NJ). The membrane was incubated for 1 h in blocking buffer (Tris-buffered saline, 0.1% Tween (TBS-T), 5% nonfat dry milk or 3% BSA) and incubated overnight at 4 °C with indicated antibodies listed in Supplementary Table 3 . Dilutions used are also listed in Supplementary Table 3 . Representative full images of key western blots are shown in full blot images in Supplementary Figs 24 and 25 . Prostate tissues In this study, we utilized tissues from clinically localized prostate cancer patients who underwent radical prostatectomy as a primary therapy between 2004 and 2006 at the University of Michigan Hospital. Samples were also used from androgen-independent metastatic prostate cancer patients from a rapid autopsy programme described previously [49] , [50] . The detailed clinical and pathological data are maintained in a secure relational database. This study was approved by the Institutional Review Board at the University of Michigan Medical School. Both radical prostatectomy series and the rapid autopsy programme are part of the University of Michigan Prostate Cancer Specialized Programme of Research Excellence Tissue Core. All tissue samples were collected with informed consent under Institutional Review Board (IRB) approved protocols at the University of Michigan. Expression and confirmation of Halo-tag fusion proteins EZH2, BMI1, RING1B, EED and subdomains were cloned into pFN19A and pFN21A vectors (Promega) in accordance to the manufacturer’s instructions. Fusion proteins were expressed in TNT SP6 High-Yield Wheat Germ Reaction (Promega) following manufacturer’s instruction or transfected into HEK293 cells for transient expression. A total of 2.0 μl of cell-free reaction containing the HaloTag fusion protein or 10 μg total proteins from HEK293 cell lysates was resolved on SDS gels and blotted using anti-Halo or indicated antibodies ( Supplementary Table 3 ) Dilutions are listed in Supplementary Table 3 . In vitro PRC2 histone methyltransferase activity assays Assays were performed according to the manufacturer’s instructions (BPS Bioscience, San Diego, CA) [51] . Purified recombinant histone H3 proteins were purchased from Active Motif (Carlsbad, CA). In brief, purified PRC2 with or without EED proteins were incubated in the reaction buffer with histone H3 proteins, together with BMI1, RING1B or control proteins, or anti-EED antibodies or control IgG. After 2 h of incubation at 37 °C, the reaction components were subjected to immunobot analysis with indicated antibodies to detect the various histone modifications. Alternatively, the purified PRC2 with or without EED proteins, together with BMI1, RING1B or control proteins, or anti-EED antibodies or control IgG, in the reaction’s buffer were incubated with the recombinant nucleosomes in pre-coated black 96-well plate at room temperature for 1 h and processed following the manufacturer’s instructions. In vitro PRC1 histone H2A E3 ubiquitin ligase activity assays Recombinant ubiquitin activating enzyme (UBE1), UbcH5c-conjugating enzyme E2, ubiquitin and Ubiquitin Conjugation Reaction Buffer Kit were purchased from Boston Biochem (Cambridge, MA). Recombinant histone H2A proteins were purchased from Millipore. EED, RING1B, BMI1 and GUS proteins were expressed in TNT SP6 High-Yield Wheat Germ Reaction and then purified. Assays were performed according to the manufacturer’s instructions and previous report [52] . In brief, H2A proteins (or reconstituted mono-nucleosomes), ubiquitin, ubiquitin activating enzyme E1 (UBE1), conjugating enzyme E2 (UBCH5C) and ligase E3 (RING1B), together with EED, BMI1 or GUS were incubated at 37 °C for 2 h, and then subjected immunoblot analysis with indicated antibodies. Dilutions are listed in Supplementary Table 3 . In vitro nucleosome assembly assays EpiMark Nucleosome Assembly Kit and recombinant Histone H2A/H2B were purchased from New England Biolabs (Ipswich, MA). Recombinant histones H3 and H4 were purchased from Active Motif. Assays were performed according to the manufacturer’s instructions and then subjected to a gel shift assay to visualize the reconstituted mono-nucleosomes. Small RNA interference Knockdowns of specific genes were accomplished by RNA interference using commercially available siRNA duplexes for EED and RING1B (Dharmacon, Lafayette, CO) [53] , [54] , [55] . At least 4 independent siRNAs were screened for knockdown efficiency against each target, and the best two siRNA duplexes were selected. Cells were plated 24 h before transfection at 50% confluence. Cells were washed twice before transfecting. Ten microliters of 20 μM siRNA duplex was diluted into 175 μl Opti-MEM I Reduced Serum Medium, and then mixed and incubated for 15 min with premixed 15 μl diluted oligofectamine (3 μl in 12 μl Opti-MEM I Reduced Serum Medium, mixed and incubated for 5 min). The siRNA/oligofectamine mixtures were then added into each well of 6-well plate with 800 μl serum-free medium. Cells were then incubated in 37 °C 5% CO 2 incubated for 4 h and then changed to 10% FBS growth medium. Transfection was repeated once after 24-h incubation. Forty-eight hours post second transfection, cells were collected for analysis. Prostate tumour xenograft model Four-week-old male SCID mice (CB.17. SCID) (Charles River Laboratory, Wilmington, MA) were used for xenograft study. A total of 2 × 10 6 DU145-Scr or DU145 EED-sh3 cells were resuspended in 100 μl of saline containing 50% Matrigel (BD Biosciences, Becton Drive, NJ) and were injected subcutaneously into both flanks of the mice ( n =9 for DU145-Scr, n =10 for DU145-EED sh3). Tumour growth was monitored weekly, and tumour volumes were estimated using the formula (π/6) ( L × W 2 ), where L =length of tumour and W =width. All procedures involving mice were approved by the University Committee on the Use and Care of Animals (UCUCA) at the University of Michigan and conform to their relevant regulatory standards. Chromatin immunoprecipitation and ChIP-Seq analysis The cells were cross-linked for 10 min with 1% formaldehyde. Cross-linking was terminated by the addition of 1/10 volume 1.25 M glycine for 5 min at room temperature followed by cell lysis and sonication, resulting in an average chromatin fragment size of 200 bp. DNA was isolated from samples by incubation with the antibody at 4 °C followed by wash and reversal of cross-linking. The ChIP-Seq sample preparation for sequencing was carried out according to the manufacturer’s instructions (Illumina). Ten to twenty nanograms of ChIP enriched DNA samples were end repaired to blunt-ended fragments using a combination of three enzymes, namely, T4 DNA polymerase, E . coli DNA polymerase I large fragment (Klenow polymerase) and T4 polynuleotide kinase (New England BioLabs, NEB). Next using Klenow fragment (3′ to 5′ exo minus; NEB) a single A-base was added to fragment ends and using Quick ligase (NEB) adaptors were ligated. The adaptor modified DNA fragments were enriched by PCR with Phusion DNA polymerase (NEB) and in that process barcoded. PCR products were size selected using 3% NuSieve agarose gels (Lonza) followed by gel extraction using QIAEX II reagents (QIAGEN). Libraries were quantified using the Bioanalyzer 2100 (Agilent), and the samples were sequenced using Illumina Hi-Seq 2000. The primer sequences for the various promoters analysed are provided in Supplementary Table 4 . ChIP-Seq data were analysed using HPeak ver. 3 (ref. 56) [56] to identify enriched regions (peak calling). Subsequently raw read window counts around TSS (transcript start site) flanking regions were summarized and visualized using Java TreeView. ChIP-Seq data sets in DU145 cells were mapped by BWA pair-end [57] . Unique pairs were selected by the XT:A:U after the removal of PCR duplicates. Top and bottom 1% chimeric pair-end tags were removed to maintain average insert size of 220–250 bp as specified by library preparations with s.d. <35 bp. On average, 80% of original data sets were retained after filtering for pair-end peak calling. The RING1B ChIP-Seq data set in mouse embryonic stem cells was downloaded from GEO (GSE23716) [35] . The original RING1B ChIP-Seq using Eed −/− mESCs (KO) data on GEO contains approximately 3.5 times more unique reads than the RING2 ChIP-Seq using Eed +/+ mESCs (WT). To reduce read imbalance between the two samples, we used a sampling approach. To be specific, we randomly sample RING1B in Eed −/− mESCs (KO) data to reduce total number of reads from 53 million to 17 million (compared with 16.8 million in Eed +/+ mESCs (WT)). The sampling process was repeated 100 times before finalized selection to reduce sampling bias. Heatmap Five kilobases around the Transcription Start Site (TSS) were considered as the gene promoter, and this region was divided into 50 bp windows. For each sample, the read count in each window is normalized over total read counts. In the heatmap, each row represents a transcript, ordered by the total coverage of the ChIP-Seq reads; each column represents a 50 bp window. Accession codes: The ChIP-Seq data has been deposited in the GEO database under accession number GSE42566 . How to cite this article: Cao, Q. et al. The Central Role of EED in the Orchestration of Polycomb Group Complexes. Nat. Commun. 5:3127 doi: 10.1038/ncomms4127 (2014).